Spatially and temporally reconfigurable assembly of colloidal crystals The self-assembly of colloidal crystals is important to the production of materials with functional optical, mechanical and conductive properties. Yet, self-assembly methods are limited by their slow kinetics and lack of structural control in space and time. Refinements such as templating and directed assembly partially address the problem, albeit by introducing fixed surface features such as templates or electrodes. A template-free method to reconfigure colloidal crystals simultaneously in three-dimensional space and time would better align work in colloidal assembly with materials applications. Here, we report a photo-induced assembly method that yields regions either filled with colloidal crystals or completely devoid of colloids. The origin of the effect is found to be electrophoresis of colloids generated by photochemistry at an indium tin oxide-coated substrate. Simple optical manipulations are applied to reconfigure these assembly and depletion regions. Thus, the method represents a new kind of template-free, reconfigurable three-dimensional photolithography. Recent efforts to produce reconfigurable colloidal assemblies have included holographic optical tweezers [1] , [2] , optically tunable electrophoretic and electrokinetic assemblies [3] , [4] , photoresponsive colloids [5] and DNA-directed assembly [6] . While powerful, these methods, respectively, are limited to small scales, require external electric fields, are not easily reversible, or have to date only yielded two-dimensional patterning. More useful for applications such as adaptive optics [7] , [8] or reconfigurable circuit elements [9] with conductive functionalities [10] would be an assembly method in which a three-dimensional colloidal crystal could not only be switched on and off in time, but could also be simultaneously controlled in space, on the micron scale, without the restriction of fixed surface features such as electrodes [11] , [12] , [13] and templates [14] , [15] , [16] . Light is an effective means for control of colloidal crystals in space and time, because its propagation is easily manipulated by commonly available microscope optics. The effect of light on colloids is typically due to radiation pressure, especially for a system with a mismatch between particle and solvent refractive index [17] . Light-induced assemblies have also been produced at the nanoscale for the specific case of cadmium telluride [18] and gold [19] nanoparticles. However, light can also be used to control the rate of chemical reactions, and therefore induce localized ion flows due to a spatial concentration gradient of reactants [20] . These ion flows create non-local electric fields that could electrophoretically assemble colloids. Here, we show results in which this conceptual idea is implemented. We induce colloidal crystallization in spatially selective regions by using light to generate a local electric field. The local electric field directs colloidal motion by coupling to charge on the particle, thereby inducing electrophoresis that leads to colloidal assembly. The local electric field is generated by illuminating an indium tin-oxide (ITO)-coated glass substrate at the base of a colloidal suspension with a 488 nm laser or an ultraviolet (UV) source. Localized illumination of the ITO coating results in motion of the particles either towards or away from the illuminated region. The assembly kinetics and structures are characterized in situ by direct visualization with a confocal laser scanning microscope. The method is fully reconfigurable, non-invasive, operates at low powers and generates structures of complex shape with sharp features. Photo-induced colloidal assembly The system studied, 1.4 μm colloidal poly(methyl methacrylate) (PMMA) stabilized with poly(12-hydroxy-stearic acid) (PHSA) and dispersed in a refractive index- and density-matched solvent of cyclohexyl-bromide (CHB) and decahydronaphthalene (decalin), is a common one for colloidal self-assembly [21] , [22] , [23] . A 200 μl solution of these colloidal particles, with 50 μM of the disassociating species tetrabutylammonium bromide (TBAB) added, was pipetted into a glass vial. The interior of the bottom of the vial had been coated with a 65 nm thick layer of indium tin oxide (ITO). When a 25 × 25 μm 2 region of the surface was illuminated with a 488 nm laser (12 W cm −2 ), accumulation of particles was observed in the vicinity of the illuminated region in about 60 s ( Fig. 1a–c ). At this condition, as in many others, the accumulation of particles was sufficient for colloidal crystal ordering ( Fig. 1e ). The greatest concentration of particles was found within the illuminated region, with modest photobleaching ( Fig. 1e ). We know that the effect of the light on the self-assembly reported in Fig. 1 is not due to optical trapping and radiation pressure, because the particles are nearly refractive index matched with the solvent ( Δn/n =0.002). The observed colloidal velocity is three orders of magnitude greater than what would be expected due to optical trapping and radiation pressure, as per a calculation using the Mie scattering theory [17] , [24] . 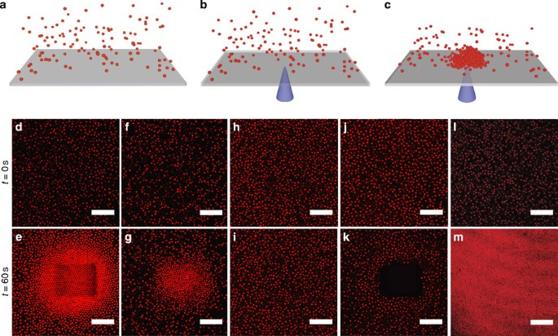Figure 1: Photo-induced colloidal assembly phenomenon. (a) PHSA-stabilized PMMA colloids (1.4 μm) at an initial volume fraction of 0.05 are initially dispersed in solution in contact with the ITO-coated glass substrate. (b) A 488 nm laser or UV light source is focused at the objective and scanned across a region of interest. (c) Particle accumulation is observed at the illuminated region. (d–m) Each image pair shows the colloidal structure before and after 60 s of excitation at 488 nm with power density 12 W cm−2(d–k) and excitation at 360 nm with power density 0.62 W cm−2(l,m). The solvent is CHB/decalin with 50 μM TBAB added (d–i,l,m) or no added TBAB (j,k). In images (d,e,j,k–m), the solution is in contact with an ITO-coated substrate; (f,g) the solution is in contact with a gold coated substrate;h,iis a control experiment in which the solution is in contact with a pure silica substrate. Scale bars, 20 μm. Figure 1: Photo-induced colloidal assembly phenomenon. ( a ) PHSA-stabilized PMMA colloids (1.4 μm) at an initial volume fraction of 0.05 are initially dispersed in solution in contact with the ITO-coated glass substrate. ( b ) A 488 nm laser or UV light source is focused at the objective and scanned across a region of interest. ( c ) Particle accumulation is observed at the illuminated region. ( d – m ) Each image pair shows the colloidal structure before and after 60 s of excitation at 488 nm with power density 12 W cm −2 ( d – k ) and excitation at 360 nm with power density 0.62 W cm −2 ( l , m ). The solvent is CHB/decalin with 50 μM TBAB added ( d – i , l , m ) or no added TBAB ( j , k ). In images ( d , e , j , k – m ), the solution is in contact with an ITO-coated substrate; ( f , g ) the solution is in contact with a gold coated substrate; h , i is a control experiment in which the solution is in contact with a pure silica substrate. Scale bars, 20 μm. Full size image The particle accumulation effect only occurred for the case of conductive or semi-conductive substrates. For example, replacing the ITO coating with gold still yielded particle accumulation ( Fig. 1f,g ). The corresponding control experiment, with illumination of a (uncoated) silica coverslip, yielded no particle accumulation ( Fig. 1h,i ). We also found that the effect requires direct contact of the ITO substrate with the colloidal solution. Specifically, when the ITO-coated substrate is flipped so that the silica side is in contact with the solution, or when the ITO layer is covered with a thin layer of deposited silica, the photo-induced motion is no longer observed. These observations, along with finite difference simulation that indicates very low temperature gradients in the system, rule out electrothermal and thermophoretic explanations of the photo-induced motion [4] , [25] . The assembly was also a sensitive function of TBAB concentration. Figure 1j,k shows that colloids were expelled from the illumination region, instead of collected, when the 50 μM of TBAB was not added to the CHB/decalin solvent mixture. Particle accumulation was also observed at other illumination wavelengths. Illumination with a mercury metal halide lamp (360 nm) yielded accumulation of particles as indicated by Fig. 1l,m . Thus, the directed assembly phenomenon is common and predicated on the coupling of electromagnetic illumination to an absorptive, conductive substrate such as ITO. Additional features of the effect, such as the solvent conditions, the particle types and the illumination wavelengths in which assembly or depletion was observed, are available. First, there is a strong effect of solvent conditions on whether or not the photo-induced effect is observed. While organic, low-dielectric constant systems, such as CHB and decalin, demonstrated significant photo-induced assembly response to electromagnetic illumination, systems of higher dielectric constants, such as dimethyl sulphoxide (DMSO) and water, showed little to no photo-induced effect. The role of solvent dielectric constant in the self-assembly of the colloids studied here has been previously established [22] , and the present effect is consistent with those previous observations. Second, in solvents in which particles do display the photo-induced effect, whether or not assembly or depletion is observed is a strong function of the kind of colloids used. The photo-induced effect was studied for PMMA colloids with various surface stabilizers and polystyrene (PS) colloids. Assembly was observed under a variety of conditions for PMMA colloids. For example, assembly occurred for different substrates illuminated (gold and ITO coating), varying wavelengths of the laser (458, 476, and 488 nm), laser powers ranging from 2.7 to 12 W cm −2 , initial volume fractions of particles varying from 0.0125 to 0.20 and particle sizes from 0.6 to 1.4 μm. All of these experiments were carried out with PHSA-stabilized PMMA colloids in CHB/decalin with a 1 mM TBAB electrolyte. Other surface-functionalized PMMA particles, such as those synthesized with the stabilizers polydimethylsiloxane (PDMS) [26] and diphenyldimethylsiloxane (DPDMS) [27] , showed depletion at the illuminated region, similar to that observed for PHSA-stabilized PMMA colloids with no TBAB. PS particles demonstrated no signs of assembly in both water and DMSO solvents of 0.1 mM TBAB under visible light excitation, whereas, under UV illumination, PS particles were found to accumulate in DMSO. Third, for particles and solvents that show the photo-induced effect, the magnitude of the effect, as indicated by the speed of the assembly and the extent and quality of the ordered structures formed, is a function of whether visible or UV light is used. With the UV illumination (360 nm), faster accumulation was observed relative to the case of visible light. Faster accumulations with UV illumination were observed for both PHSA-stabilized PMMA colloids and for PS particle suspensions. For these cases, PMMA particle suspensions were prepared in a 1 mM TBAB solution of CHB/decalin. Three-dimensional structure of the assembled crystals The photo-induced effect yields finite-thickness quasi-2D colloidal crystals. At steady-state, and at the laser power densities studied, the penetration depth of the accumulation was about 10 μm, resulting in a stacking of about five crystalline layers ( Fig. 2a,b ). The 3D structure of the crystal, as rendered by image analysis of CLSM volumes, showed close-packed ordering with some defect structure ( Fig. 2c,d ). The local number density ( N/V ) of colloids was as large as 0.95 particles μm −3 at the ITO substrate at the largest power density studied (12 W cm −2 ). The periodic variation in particle density apparent in Fig. 2e is further evidence of the layered structure, consistent with a colloidal crystal. The effect of the light on the self-assembly is significant. As the power is changed from 12 to 2.7 W cm −2 , the near-wall particle number density of the sample decreases from 0.95 to 0.46 particles μm −3 . Both self-assemblies, however, have crystalline structure. Under these conditions, the near-wall crystalline volume fractions (within the first three layers) are 47 and 34%, respectively. These values are consistent with that of the disorder to order transition boundary expected for the system of charged PHSA-stabilized PMMA colloids. The theoretical phase transition boundary was determined to be ϕ =0.36, given the measured Debye screening length (95 nm) and the colloid zeta potential (−9 mV) [28] . 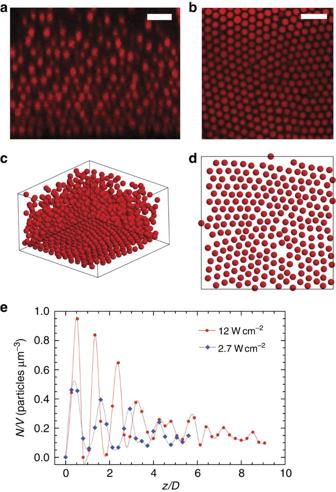Figure 2: Three-dimensional structure of the photo-induced assembly. The particle and solvent conditions are as inFig. 1eand the illumination time is 120 s. (a) Image acquired perpendicular to the ITO coverslip shows accumulation of multiple layers of colloids above the region of illumination. Scale bar, 5 μm. (b) Image of the same structure acquired at the ITO coverslip. Scale bar, 5 μm. (c) 3D rendering of CLSM-derived colloid centroids shows crystalline structure; colloid centroids were identified by image processing; (d) Rendering of the crystalline layer closest to the coverslip, which shows hexagonal ordering, with some defect structure. (e) Particle number density (N/V) of the assembly is a function of distance from the substrate and laser power density. Figure 2: Three-dimensional structure of the photo-induced assembly. The particle and solvent conditions are as in Fig. 1e and the illumination time is 120 s. ( a ) Image acquired perpendicular to the ITO coverslip shows accumulation of multiple layers of colloids above the region of illumination. Scale bar, 5 μm. ( b ) Image of the same structure acquired at the ITO coverslip. Scale bar, 5 μm. ( c ) 3D rendering of CLSM-derived colloid centroids shows crystalline structure; colloid centroids were identified by image processing; ( d ) Rendering of the crystalline layer closest to the coverslip, which shows hexagonal ordering, with some defect structure. ( e ) Particle number density ( N / V ) of the assembly is a function of distance from the substrate and laser power density. Full size image Kinetics of the photo-induced assembly The photo-induced assembly process occurs rapidly. The characteristic time for assembly is about 60 s ( Fig. 3a–f ). On laser exposure, particles are displaced from the suspension into the illuminated region, as also shown in Supplementary Movie 1 . Particles begin to concentrate a few seconds after the ITO-coated surface is exposed to the laser ( Fig. 3b ), until a crystalline structure is formed. Accumulated particles display a close-packed crystal ordering ( Fig. 3e ). For initial volume fractions studied ( ϕ 0 =0.0125–0.20), the photo-induced volume fraction monotonically increases with time and reaches a steady state ( Fig. 3g ). From Fig. 3g , a characteristic time for crystallization, t c , was defined as the time for the assembly to reach 99% of its steady-state volume fraction. 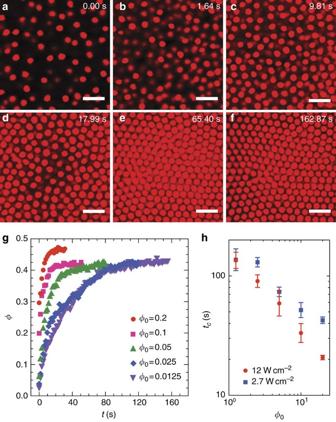Figure 3: Kinetics of assembly under optical field excitation. (a–f) Time lapse images of PMMA particles (ϕ0=0.05) concentrating in the 25 × 25 μm2region that was illuminated. The particle and solvent conditions are as inFig. 1e. Scale bar, 5 μm. (g) Particle volume fraction,ϕ, monotonically increases until it reaches steady state. (h) Quantification of the critical concentration time,tc, shows that time for accumulation decreases with increasing laser power density and initial volume fraction. The error bars indicate s.d. Figure 3h shows that t c decreases with increasing ϕ 0 and laser power. Figure 3: Kinetics of assembly under optical field excitation. ( a – f ) Time lapse images of PMMA particles ( ϕ 0 =0.05) concentrating in the 25 × 25 μm 2 region that was illuminated. The particle and solvent conditions are as in Fig. 1e . Scale bar, 5 μm. ( g ) Particle volume fraction, ϕ , monotonically increases until it reaches steady state. ( h ) Quantification of the critical concentration time, t c , shows that time for accumulation decreases with increasing laser power density and initial volume fraction. The error bars indicate s.d. Full size image The sedimentation dynamics was used to infer a particle velocity from measurements of t c, as shown in Supplementary Fig. 1 . The photo-induced particle velocity (1,000 μΜ TBAB and 12 W cm −2 ) was found to be 0.28±0.02 μm s −1 , independent of the initial volume fraction. The decrease in t c with ϕ 0 is a consequence of the faster filling of the assembly region due to the greater local availability of colloids at higher ϕ 0 . That is, at low ϕ 0 , it takes longer to crystallize the near-wall layer because the accumulating colloids must be drawn from a larger reservoir. Effect of TBAB concentration on the photo-induced assembly The effect of light on assembly was a strong function of TBAB concentration. 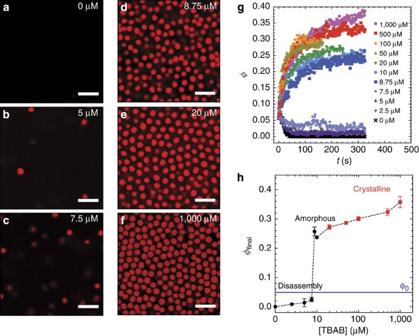Figure 4: Influence of the TBAB concentration on the photo-induced effect. Images are acquired 150 s after illumination and the initial colloid volume fraction is 0.05. For these colloids, the particle zeta potential is a known function of TBAB concentration. (a–c) Images show PMMA colloid migration away from the illuminated region, thereby generating a void region of low colloid concentration. (d–f) Images show PMMA colloid migration towards the illuminated region, thereby leading to concentration and assembly. Scale bar, 5 μm. (g) For TBAB concentrations under 7.5 μM,ϕdecreases from its initial volume fraction, indicating depletion of particles within the region of interest. Above 7.5 μM TBAB, the volume fraction increases monotonically to a higher final volume fraction. (h) Final volume fraction values are extracted fromgand plotted against their TBAB concentrations. There is a distinct transition between 7.5 and 8.75 μM TBAB; depletion is observed below this transition and assembly is observed above. The error bars indicate s.d. Figure 4 shows a transition from depletion to assembly with varying [TBAB]. As TBAB concentration is varied from 0 to 1,000 μM, reversal of the photo-induced effect occurs abruptly between TBAB concentrations of 7.5 and 8.75 μM. Below the threshold condition of 7.5 μM, depletion of particles from the illuminated region was observed ( Fig. 4a–c ). The kinetics of the depletion effect are in Supplementary Movie 2 . Between salt conditions of 8.75 and 10 μM, the system demonstrated a weak driving force for assembly, as evidenced by the observation that the accumulation effect was not strong enough to generate a colloidal crystal. A disordered, liquid structure was instead observed ( Fig. 4d ). For TBAB concentrations greater than 20 μM, the steady-state assemblies generated were crystalline. Increase in salt concentrations led to a small increase in assembly volume fraction in this range of TBAB concentration. This small change is due to the crystalline structure having smaller particle separations at higher salt concentrations, due to the changing Debye length. Figure 4: Influence of the TBAB concentration on the photo-induced effect. Images are acquired 150 s after illumination and the initial colloid volume fraction is 0.05. For these colloids, the particle zeta potential is a known function of TBAB concentration. ( a – c ) Images show PMMA colloid migration away from the illuminated region, thereby generating a void region of low colloid concentration. ( d – f ) Images show PMMA colloid migration towards the illuminated region, thereby leading to concentration and assembly. Scale bar, 5 μm. ( g ) For TBAB concentrations under 7.5 μM, ϕ decreases from its initial volume fraction, indicating depletion of particles within the region of interest. Above 7.5 μM TBAB, the volume fraction increases monotonically to a higher final volume fraction. ( h ) Final volume fraction values are extracted from g and plotted against their TBAB concentrations. There is a distinct transition between 7.5 and 8.75 μM TBAB; depletion is observed below this transition and assembly is observed above. The error bars indicate s.d. Full size image The effect of TBAB on the photo-induced assembly was quantified by measuring the local, near-wall colloid volume fraction as a function of time. Consistent with qualitative observations, ϕ decreases relative to the initial volume fraction for [TBAB]<7.5 μM and increases for [TBAB]>8.75 μM ( Fig. 4g ). Near steady-state volume fractions were reached for all conditions. By plotting the final volume fraction measured at each TBAB condition, the abrupt transition from colloidal depletion (at low TBAB concentration) to assembly (at high TBAB concentration) is apparent ( Fig. 4h ). The abruptness of the change, and the fact that it occurs at a finite TBAB concentration, argues against a role of the changing Debye length in this transition. Rather, we will show that the abrupt change at ~8 μM TBAB is more likely due to the effect of [TBAB] on the colloid zeta potential. Taken together, these results constrain possible mechanisms of the photo-induced assembly. To summarize, the mechanism must be consistent with local colloid motion of ~0.3 μm s −1 induced when a metallic or semiconducting substrate is illuminated with a 488 nm visible light at a power of 12 W cm −2 (for the UV case, the corresponding measured velocity is 1.8±0.3 μm s −1 at a power of 0.62 W cm −2 ); near refractive index matching ( Δn/n =0.002) of the colloids and solvent; requirement that the semiconducting or metallic substrate is in direct contact with the colloidal solution; change from colloidal depletion to assembly in the region of illumination at ~8 μM as TBAB concentration is varied between 0 and 1,000 μM. 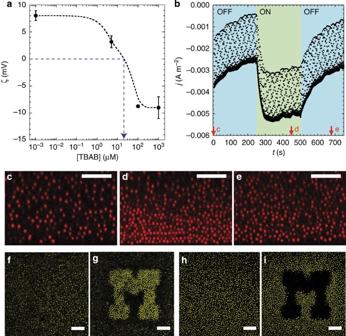Figure 5: Electrophoretic origin of the photo-induced assembly mechanism. (a) Zeta potential values of PHSA-stabilized PMMA colloids undergo a change in sign at about 20 μM added TBAB. The dotted curve is a line to guide the eye. The error bars indicate s.d. (b) When the photo-induced effect is generated in a cell with electrodes, the measured current exhibits a rapid change as a direct response of the UV light being turned on and off. This experiment was carried out with PHSA-stabilized PMMA colloids prepared at 5% volume fraction and 1,000 μM concentration of TBAB. (c–e) CLSM images corresponding to the times marked inb. Images taken perpendicular to the coverslip show that the effect of light on the particle assembly is temporally correlated with changes in current density due to the illumination. Scale bar, 15 μm. (f–i) Because the current density is produced only in the illuminated region, the photo-induced assembly and depletion effects can be achieved when complex shapes are illuminated by the light, as is possible by, for example, using the optics of the scanning microscope. (f,g) Before and after images of colloidal assembly show accumulation of particles in the illuminated region of complex shape. The colloidal solution was prepared at 5% initial volume fraction with 1,000 μM TBAB in CHB/decalin. (h,i) Before and after images of colloidal depletion show depletion of particles within the illuminated region of complex shape. The initial colloidal volume fraction was 10%, and the solvent was pure CHB/decalin. Scale bars, 20 μm. Mechanism of the photo-induced colloidal crystallization Figure 5 suggests a mechanism consistent with these findings. Independent measurements of the zeta potential of the PMMA colloids ( Fig. 5a ) show a remarkable coincidence between the sign of the measured colloid zeta potential (which reverses at ~20 μM TBAB) and the switch of the effect from depletion to assembly (which occurs at ~8 μM TBAB). This sensitivity of PMMA colloid zeta potential to TBAB concentration, including a change in the sign of the zeta potential, is consistent with the literature [29] . The coincidence of the assembly/depletion transition and the change in sign of the zeta-potential suggest that the photo-induced assembly effect is induced by light-induced electrophoresis of the colloids. This mechanism would imply the existence of an electric field in the system. While no electrode geometry has been fabricated into the system, the metallic surface itself is potentially reactive [3] , [30] . If the surface were a substrate for chemical reactions, the resulting depletion in chemical species at the substrate would result in an ion flow normal to the illuminated region of the substrate. This ion flow will produce a current that yields an electric field of magnitude , where j is the measured current density (per illuminated area) and λ 0 is the conductivity of the solution [31] . Thus, if photo-induced electrophoresis is the mechanism for the observed directed assembly, then a current ought to be set up in the system when light illuminates the ITO substrate. The current itself is quite small because of the small illumination area (~1.8 × 10 4 μm 2 in most cases). The magnitude and direction of the current should be consistent with the magnitude and sign of the colloid zeta-potential. Ion flows of the kind hypothesized here have previously been reported for non-aqueous solvents [32] . Figure 5: Electrophoretic origin of the photo-induced assembly mechanism. ( a ) Zeta potential values of PHSA-stabilized PMMA colloids undergo a change in sign at about 20 μM added TBAB. The dotted curve is a line to guide the eye. The error bars indicate s.d. ( b ) When the photo-induced effect is generated in a cell with electrodes, the measured current exhibits a rapid change as a direct response of the UV light being turned on and off. This experiment was carried out with PHSA-stabilized PMMA colloids prepared at 5% volume fraction and 1,000 μM concentration of TBAB. ( c – e ) CLSM images corresponding to the times marked in b . Images taken perpendicular to the coverslip show that the effect of light on the particle assembly is temporally correlated with changes in current density due to the illumination. Scale bar, 15 μm. ( f – i ) Because the current density is produced only in the illuminated region, the photo-induced assembly and depletion effects can be achieved when complex shapes are illuminated by the light, as is possible by, for example, using the optics of the scanning microscope. ( f , g ) Before and after images of colloidal assembly show accumulation of particles in the illuminated region of complex shape. The colloidal solution was prepared at 5% initial volume fraction with 1,000 μM TBAB in CHB/decalin. ( h , i ) Before and after images of colloidal depletion show depletion of particles within the illuminated region of complex shape. The initial colloidal volume fraction was 10%, and the solvent was pure CHB/decalin. Scale bars, 20 μm. Full size image To test this hypothesis, we performed the following experiment. For a solution of 5 vol% particles in CHB/decalin with 1,000 μM TBAB, the current density, j , was measured as UV illumination (360 nm, 0.62 W cm −2 ) was turned on and off ( Fig. 5b ). We found a significant change in the current density as the UV light was switched on and off. Simultaneously, CLSM images were collected ( Fig. 5c–e ). The results show that the application of light coincides with both change in the current density and the observation of assembly. Additional details are also consistent with the mechanism: First, the negative zeta potential (at 1,000 μM TBAB) is in accord with the observation of colloidal motion towards the illuminated electrode at this condition. Specifically, particle motion in this direction indicates that the illuminated electrode is the anode, consistent with the negative sign of the measured cathodic current, as plotted in Fig. 5b (ref. 31 ). Second, the up and down motion of the microscope’s optical scanner is observable in the current density ( Fig. 5b ), consistent with an effect of visible light on accumulation. Third, the magnitude of the colloidal velocity predicted from the electric field is consistent with direct measurements of UV-induced velocities. Further details of these observations are given in Supplementary Note 1 . The photo-induced assembly, therefore, occurs due to an electric field generated by a light-induced current. Similar types of photo-induced current modulation have been observed in the past [3] , but never in the absence of an externally applied electric field and fixed electrodes. Here, instead, the electric field is generated internally. It is this internally generated field, induced by light alone, that allows the simultaneous spatial and temporal control of the assembly without need for other hardware, such as templating or electrodes. We point to two potential origins of the light-induced chemistry. The light could catalyse a reaction of dissolved species, such as residual water, oxygen, or surfactants such as TBAB at the ITO substrate; these redox reactions would drive a current that would induce an electric field; or, the light-induced ionization of dissolved species, such as TBAB, could create a concentration gradient within the solution, spontaneously setting up an electric field and thereby generating electrodiffusiophoresis [33] . Both mechanisms are consistent with the observation that the photo-induced motion requires illumination of a semiconducting or metallic substrate that is in direct contact with the colloidal solution. The fact that the phenomenon requires a light/reactive substrate interaction means that the effect is extremely localized in space and time. Figure 5f–i shows application of this understanding to create complex shapes of colloids. A 405 nm laser scanned this intricate design, drawn as a region-of-interest (ROI) by using the microscope’s optical scanner. The experimental conditions of the assembly ( Fig. 5f,g ) and the depletion ( Fig. 5h,i ) are in the figure legend. The kinetics of these reconfigurable colloidal assemblies are available in Supplementary Movies 3,4 . We find that colloids rapidly assemble and deplete within a few seconds of illumination to form structures with sharp features and well-defined boundaries. The definition of these features and boundaries are as good for the case of depletion as for assembly. Both kinds of structures created are fully reversible. The results indicate the method’s rapidity, reversibility and spatial specificity for producing 3D regions of colloidal ordering and depletion. With these characteristics, the photo-induced electrophoretic method has broad application for new materials comprising reconfigurable assemblies, especially for the template free, spatially selective assembly of 3D colloidal crystals. Colloidal system and sample preparation The colloidal particles used for the photo-induced assembly were PHSA-stabilized PMMA ( D =1.40 μm, 5.6% polydispersity). Particles were dispersed in a refractive index- and density-matched solvent mixture of 66 vol% cyclohexyl-bromide (CHB) and 34 vol% decahydronaphthalene (decalin). Experiments were carried out in suspensions of initial volume fraction, ϕ 0 , varying from 0.0125 to 0.20 and added TBAB concentration varying from 0 to 1,000 μM. Two hundred microlitres of colloidal suspension was dispensed into a specimen vial with a cylindrical geometry ( D =10 mm, H =1.25 mm). ITO-coated microscope coverslips ( d ~0.170 mm) were used as the bottom surface of the vial, with the ITO coating facing inwards. The ITO coating was ~65 nm thick with ~500 Ω sq. sheet resistance −1 (ZC & R Coatings, Inc.). In one set of experiments, a gold coating was used instead of the ITO coating (~15 nm thick with ~7.5 nm chrome layer, Denton Vacuum). Light illumination Two different light sources were used for the photo-induced assembly. First, 488 nm laser light was focused at the ITO-coated coverslip using a 100X oil immersion objective lens ( NA =1.40). The laser power was delivered by using a confocal laser scanning microscope (CLSM, Leica TCS SP2 or Nikon A1R), in which a pointwise scan of the region (25 × 25 μm 2 ) was performed with a duty cycle of 66%. The laser power density varied from 2.7 to 12 W cm −2 (Optical power meter 1916-C, detector 818-ST, Newport). Second, a UV light source (Leica EL6000, Mercury metal halide bulb, 360 nm) was used for illumination in some cases. This radiation was projected onto a circular region ( D =150 μm) with a mean flux of 0.62 W cm −2 (UV meter 306, OAI). Another UV light source (Nikon A1R stimulation scan, 405 nm) was used to scan a ROI of a complex shape. Confocal microscope imaging conditions CLSM was used to characterize the kinetics and structure of the photo-induced assembly (100X objective, NA =1.40). For the assembly kinetics, time series of 100–150 frames (512 × 512 pixels) with spatial resolution of 49 nm pixel −1 were collected at a frame rate of 1.6 s. For the assembly structure, 3D image volumes of 25 × 25 × 10 μm 3 were acquired at the voxel size of 49 × 49 × 46 nm 3 . Centroidal coordinates of all particles were determined by methods discussed in Crocker et al. and characterized in Dibble et al. [34] , [35] The image analysis yielded centroidal coordinates resolved at the scale of ±35 nm in the object plane and ±45 nm in the axial direction. From these centroidal coordinates, we characterized the crystallization kinetics by determining the number of particles identified at each time frame. The structure of the ordered array was visualized by rendering the centroidal coordinates. The particle number density as a function of height above the ITO-coated substrate was determined by evaluating the number of particles in slices of size 21 × 21 × 0.4 μm 3 . The particle volume fractions of the crystals were calculated from the three layers closest to the coverslip. For the analysis of Figs 3 , 4 , the near-wall volume fraction was that of the close-packed layer at the coverslip. The ROI stimulation method of CLSM (Nikon A1R, 100 × oil objective, NA =1.49) was used to create assembly and depletion structures of complex shapes. Simultaneous imaging (561.6 nm) and scanning (405 nm) were done with a resonant scanner at a frame rate of 0.067 s. Stimulation area was defined by the ROI designed as a specific shape on the confocal software. Images (512 × 512 pixels) were collected at a spatial resolution of 0.249 μm pixel −1 . Photo-induced velocity measurements The laser-induced colloidal velocity was calculated by adapting an analysis available for sedimentation kinetics [28] . The details of the analysis method are further described in Supplementary Note 2 . The UV-induced colloidal velocity was measured from tracking the colloidal motion. Here, the distance that the particle travelled within two consecutive images was measured and divided by the frame rate (0.815 s) to calculate the particle velocity. From a series of ~200 images, sequential images were extracted and analysed to determine the average velocity. Zeta potential and current measurements Zeta potential and current measurements were made in the DC electric field device described by Shah et al . [32] Zeta-potential measurements were carried out in 1.25 vol% particle suspensions with TBAB concentrations varying from 0 to 1,000 μM. Particle mobility was tracked in planes perpendicular to the coverslip as a constant current was applied with the potentiostat (Autolab PGSTAT 128N) across the solution. Images were collected at 0.815 s per frame. Given the measured mobility, the electric field set up by the applied current, solvent properties ( ε =5.962, μ =0.0025 Pa s) and the electrolyte properties ( Λ 0 TBA+ =6.5 cm 2 S mol −1 and Λ 0 Br− =14.5 cm 2 S mol −1 ) [29] , zeta-potentials were computed by using the method of O’Brien and White [36] . Similarly, the current density changes within the suspension were measured as light was turned on and off. UV illumination (360 nm peak wavelength) at 0.62 W cm −2 was applied. The potentiostat was used to measure the current density variations under a constant zero potential (current detection range ~100 pA). How to cite this article: Kim, Y. et al. Spatially and temporally reconfigurable assembly of colloidal crystals. Nat. Commun. 5:3676 doi: 10.1038/ncomms4676 (2014).